Origami lithium-ion batteries There are significant challenges in developing deformable devices at the system level that contain integrated, deformable energy storage devices. Here we demonstrate an origami lithium-ion battery that can be deformed at an unprecedented high level, including folding, bending and twisting. Deformability at the system level is enabled using rigid origami, which prescribes a crease pattern such that the materials making the origami pattern do not experience large strain. The origami battery is fabricated through slurry coating of electrodes onto paper current collectors and packaging in standard materials, followed by folding using the Miura pattern. The resulting origami battery achieves significant linear and areal deformability, large twistability and bendability. The strategy described here represents the fusion of the art of origami, materials science and functional energy storage devices, and could provide a paradigm shift for architecture and design of flexible and curvilinear electronics with exceptional mechanical characteristics and functionalities. Deformable energy storage devices are emerging as indispensable components for unconventional electronic devices that are able to survive significant degrees of deformation, mainly bending and stretching, with strain levels much greater than 1%. Examples include flexible displays [1] , [2] , [3] , [4] , stretchable circuits [5] , hemispherical electronic eyes [6] and the recently developed epidermal electronics [7] . The energy storage devices present a significant challenge for developing a robust deformable system since they must be seamlessly integrated with deformable functional devices and energy supplies with similar mechanical characteristics, including linear deformability (that is, stretchability and compressibility), bendability and twistability. For bending deformation, many thin-film-based energy solutions such as supercapacitors [8] , [9] , [10] , [11] and batteries [10] , [12] , [13] , [14] , [15] , [16] have been developed that take advantage of the inherently small strains (usually less than 1%) near the mechanical neutral planes [17] . Recently, a handful of efforts have been undertaken to develop stretchable energy sources. Stretchable supercapacitors using buckled carbon nanotube (CNT) macrofilms as electrodes [18] , [19] and CNT-coated porous conductive textiles [20] have been developed with over 30% stretchability. Stretchable lithium-ion batteries (LIBs) with over 100% stretchability and 50% areal coverage have been demonstrated that used serpentine interconnects and that were packaged by elastomeric materials [21] . To date, approaches that simultaneously achieve a high level of deformability (including linear stretching and compression, bending, twisting and their combinations in any order) with large areal coverage that are compatible with commercially available manufacturing technologies have not been demonstrated. These attributes represent desired requirements to fully integrate energy storage devices with deformable electronics to reach system-level deformability in realistic applications. Origami-based approaches represent a potentially game-changing alternative to enable deformability over existing methods that use elastomeric materials and mechanically designed structures such as buckling and serpentine shapes. Using origami, the ancient art of paper folding, compact deformable three-dimensional structures can be created from two-dimensional sheets through high degrees of folding along predefined creases. Origami-based approaches have recently been pursued in several practical applications, including a foldable telescope lens [22] for space exploration and in heart stents [23] . In this paper, we report an approach to enable origami LIBs with the attributes of extreme mechanical deformability, including significant system-level linear and areal deformability, large twistability and bendability, and up to 74% areal coverage. Furthermore, commercially standard packaging technologies are used in the origami LIBs, which when combined with other deformable electronic devices may lead to direct practical applications. 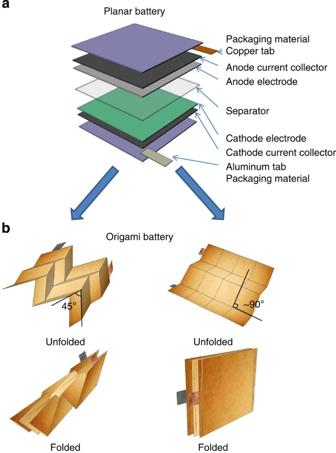Figure 1: Concept of origami lithium-ion batteries. (a) Exploded view of the multilayer structure of conventional LIBs in the planar state. (b) Two examples of origami LIBs using Miura folding. The lower left pictures refer to 45° Miura folding in the unfolded and folded states, showing that it can be completely compressed in one direction. The lower right pictures refer to 90° Miura folding in the unfolded and folded states, showing that it can be completely collapsed in biaxial directions. Battery design using Miura folding Figure 1 illustrates the origami LIB concept. Starting from conventional planar LIBs ( Fig. 1a ) consisting of many layers, including current collectors, anode and cathode, separator and packaging, the origami LIBs were realized by folding these layers based on specific origami patterns of Miura-ori [24] . In the Miura-ori pattern, shown in Fig. 1b , many identical parallelogram faces are connected by ‘mountain’ and ‘valley’ creases. Depending on the difference in angles between adjacent ‘mountain’ and ‘valley’ creases, the Miura-ori can be either almost completely compressible in one direction (lower left of Fig. 1b , and referred to as ‘45° Miura folding’ hereafter) or collapsible in two directions (lower right of Fig. 1b , and referred to as ‘90° Miura folding’ hereafter). Despite the overall high level of deformability that can be realized, the parallelogram faces themselves remain undeformed because the folding and unfolding of the creases maintains the faces in a rigid configuration. This class of origami pattern is appropriately called rigid origami, where deformability at the system level is prescribed by the creases, while the base or substrate materials making the origami pattern do not experience large strain except at the creases. Figure 1: Concept of origami lithium-ion batteries. ( a ) Exploded view of the multilayer structure of conventional LIBs in the planar state. ( b ) Two examples of origami LIBs using Miura folding. The lower left pictures refer to 45° Miura folding in the unfolded and folded states, showing that it can be completely compressed in one direction. The lower right pictures refer to 90° Miura folding in the unfolded and folded states, showing that it can be completely collapsed in biaxial directions. Full size image To achieve good foldability and electrical conductivity at the creases after cyclic folding and unfolding, we adopted CNT-coated paper as the current collectors on which we deposited active material layers [10] , [25] . Supplementary Fig. 1a,b show the optical and scanning electron micrographs (SEMs) of this paper current collector, which was produced by coating thin and porous laboratory Kimwipes (Kimtech Science, Kimberly-Clark) with CNT layers of ~40 μm thickness after drying. The electrical resistance of this paper current collector on each side was about 5 Ω per square. LiCoO 2 (LCO, Sigma-Aldrich) and Li 4 Ti 5 O 12 (LTO, MTI Corp.) were chosen as active materials for the cathode and anode electrodes, respectively. Conventional slurries of these materials were prepared and used to coat the CNT-coated paper current collectors. The battery cell was assembled in an argon-filled glovebox using 1 M LiPF 6 in EC:DMC:DEC(4:2:4) (MTI Corp), polypropylene (Celgard 2500) and aluminized polyethylene (PE) (Sigma-Aldrich) as electrolyte, separator and packaging materials, respectively. Then the assembled battery cell (shown in Supplementary Fig. 1c ) was folded using the desired origami patterns ( Fig. 1 ) in an ambient environment. The thickness of the assembled LIB cell was 380 μm. Supplementary Fig. 1d–g provides optical and SEM images of as-coated anode and cathode electrodes in the regions of a crease, showing that there were no apparent cracks or delamination of active materials from the electrodes, as compared with the planar regions. Moreover, it was verified that the electrical resistance of the electrodes before and after folding in the origami pattern (without packaging) remained unchanged. Galvanostatic charge and discharge tests were performed using a battery testing unit (Arbin Instruments). Details appear in the Methods section. 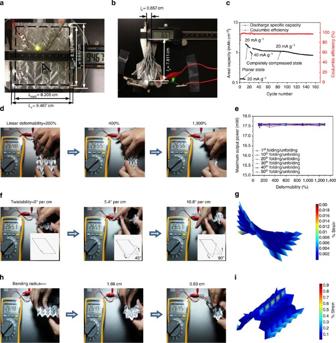Figure 2: Characteristics of the origami lithium-ion batteries using 45° Miura folding. (a) Photograph of the origami battery in the completely unfolded state, where the battery was used to power a light-emitting diode (LED). The size of the origami battery isLx×Lyand the active electrodes cover the area ofLxact×Lyact. The areal coverage is 74%. (b) Photograph of the origami battery operating a LED in its completely compressed state. The size of the battery islx×ly. (c) Capacity retention (left axis, black) and coulumbic efficiency (right axis, red) as a function of cycle number for two current densities, 20 and 40 mA g−1. (d) Photograph of linear deformation (that is, folding and unfolding) of an origami LIB while it was connected to a voltmeter. (e) Maximum output power of the origami LIB as a function of linear deformability over 50 cycles of folding and unfolding. (f) Twisting an origami LIB while it was connected to a voltmeter. (g) Finite element results of the strain contour of a 45° Miura pattern subjected to twisting with twisting angle of 90° per unit cell. (h) Bending an origami LIB while it was connected to a voltmeter. (i) Finite element results of the strain contour of a 45° Miura pattern subjected to bending with bending radius of two unit cell. Electrochemical and mechanical characteristics Figure 2 shows the results for the LIBs using 45° Miura folding. Figure 2a,b shows the pictures of the planar and completely compressed configurations, respectively. The dotted black lines highlight the area of anode and cathode electrodes, which provides over 74% areal coverage. Electrochemical properties of the LIB in its planar state (for the 1 st , 5 th and 10 th cycles) and completely compressed state (for the 30 th , 50 th , 100 th and 150 th cycles) under a current density of 20 mA g −1 are shown in Supplementary Fig. 2a . The areal capacity for the planar and completely compressed states as a function of charge rate was examined by performing galvanostatic cycling under two current densities ( Fig. 2c ). At a current rate of 20 mA g −1 , the areal capacity was about 0.2 mAh cm −2 for the first 11 cycles when the origami battery was in its planar unfolded state, and increased to 1.4–2.0 mAh cm −2 for the next 10 cycles when the origami battery was completely compressed. When the current rate was increased to 40 mA g −1 for the next five cycles, the areal capacity remained at 0.8–1.0 mAh cm −2 . When the current density was reduced back to the initial level of 20 mA g −1 , the areal capacity nearly recovered to 1.3–1.4 mAh cm −2 and remained at >1.0 mAh cm −2 for up to 110 cycles, which indicates reasonably good areal capacity. The observed decrease in the capacity after many cycles (that is, two months of continuous charging/discharging) may be attributed to the factors related to leakage in the present aluminized PE packaging, which can be improved with better seals. The present areal capacity for the completely compressed state of 1.0–2.0 mAh cm −2 could be further increased by adding more active materials (for example, LTO and LCO) to obtain thicker electrodes. However, such a modification might reduce the rate capacity and could also lead to difficulty in folding, and higher localized strain at the creases. Figure 2: Characteristics of the origami lithium-ion batteries using 45° Miura folding. ( a ) Photograph of the origami battery in the completely unfolded state, where the battery was used to power a light-emitting diode (LED). The size of the origami battery is L x × L y and the active electrodes cover the area of L x act × L y act . The areal coverage is 74%. ( b ) Photograph of the origami battery operating a LED in its completely compressed state. The size of the battery is l x × l y . ( c ) Capacity retention (left axis, black) and coulumbic efficiency (right axis, red) as a function of cycle number for two current densities, 20 and 40 mA g −1 . ( d ) Photograph of linear deformation (that is, folding and unfolding) of an origami LIB while it was connected to a voltmeter. ( e ) Maximum output power of the origami LIB as a function of linear deformability over 50 cycles of folding and unfolding. ( f ) Twisting an origami LIB while it was connected to a voltmeter. ( g ) Finite element results of the strain contour of a 45° Miura pattern subjected to twisting with twisting angle of 90° per unit cell. ( h ) Bending an origami LIB while it was connected to a voltmeter. ( i ) Finite element results of the strain contour of a 45° Miura pattern subjected to bending with bending radius of two unit cell. Full size image The mechanical characteristics of the fully charged LIBs using 45° Miura folding were examined. As shown in Fig. 2d , under folding and unfolding, the output voltage remained steady at 2.65 V (same as the highest voltage shown in Supplementary Fig. 2a for the fully charged LIB), even up to 1,340% linear deformability with respect to its completely compressed state. Supplementary Movie 1 shows the dynamic process of the linear deformation. Electrochemical impedance spectroscopy (EIS) studies were performed during the first discharge cycle before and after the mechanical deformation, and no significant changes in the impedance were found before and after mechanical deformation ( Supplementary Fig. 2b,c ). The linear deformability ∈ deformability is defined by using the dimensions marked in Fig. 2a,b as, for the x direction, and for the y direction. l x and l y are the dimensions for the completely compressed state ( Fig. 2b ), and L x and L y are the dimensions for the unfolded states, with the extreme case being the planar state shown in Fig. 2a . In other words, the deformability is defined for the unfolded states using the completely compressed state as the reference. This definition allows for the quantification of the extreme capacity for deformation in Miura folding, namely, from the completely compressed state to the planar state through unfolding, and vice versa, from the planar state to the completely compressed state through folding. Using the measured dimensions shown in Fig. 2a,b , the origami LIB with 45° Miura folding demonstrated up to 1,340% linear deformability in the x direction, going from the completely compressed state to the planar state. The areal deformability ε Areal can be correspondingly defined as , and was found to reach, 1,670%. These levels of linear and areal deformability significantly surpass those previously reported in stretchable interconnects, devices, supercapacitors and batteries. Figure 2e shows the maximum output power of the origami battery as a function of linear deformability, , under different cycles of linear deformation. Here the internal resistance of the battery was about 79 Ω. Up to a linear deformability of 1,340% and over 50 linear deformation cycles, the output power was quite stable and showed no noticeable decay. This stable performance is attributed to good bonding quality between the electrodes and CNT-coated paper current collectors, the unchanged electrical resistance of the CNT-coated paper current collectors on linear deformation and the vanishing deformation at the parallelogram faces for rigid origami. The output power of 17.5 mW is sufficient to operate commercial light-emitting diodes (LEDs). As shown in the supporting information ( Supplementary Fig. 3a–c and Supplementary Movie 2 ), LEDs driven by this LIB do not show noticeable dimming on cyclic linear deformation, even for a higher deformation rate (~0.2 m s −1 ). Figure 2f shows the optical photograph of the same origami battery subjected to torsion after tension; the dynamic process is shown in the Supplementary Movie 1 . It is clear that the origami battery using 45° Miura folding can bear large torsions of up to 10.8°cm −1 twisting angle without degradation of the output voltage. Supplementary Fig. 4 shows the maximum output power of the battery as a function of twisting angle for various twisting cycles in which a similar stability to that for tension was repeatedly observed. It is relevant to note that for a rigid origami there are ( n− 3) degrees of freedom with n as the number of edges at one vertex [26] , [27] , which gives only one degree of freedom for the Miura pattern ( n =4). Therefore, an ideally rigid Miura-folded device can only bear linear deformation, and torsion will cause strain on those parallelogram faces. Finite element analysis (FEA) was conducted by using a recently developed approach, and the strain contour is shown in Fig. 2g for 10° per unit cell twisting angle, where the size of a unit cell is the shortest length of one parallelogram face. It is clear that the strain for most of the area was vanishingly small with strain levels on the order of 0.001%. FEA is briefly provided in the supporting information and the details will be reported in a separate paper. After tension and torsion, the same device was subjected to bending, as shown in Fig. 2h . Similar mechanical robustness was observed as for tension and torsion: the origami battery could be wrapped around an index finger (with bending radius of about 0.83 cm) without a large change in the output voltage. Supplementary Fig. 5 shows the maximum output power versus bending radius under different bending cycles, and the power stability was repeatedly observed. Bending is similar to twisting as it causes strain on the parallelogram faces. Figure 2 (i) shows the strain contour of a bent Miura folding pattern with a bending radius of two unit cells, showing that the strain was again quite small—on the order of 0.1%. In addition to the 45° Miura folding pattern that can achieve significant linear deformability and bear tension, torsion and bending, a Miura folding pattern with 90° angle (lower right panel of Fig. 1 ) was also utilized. This folding can be completely collapsed in biaxial directions and thus can reach very high areal deformability. As shown in the supporting information ( Supplementary Fig. 6 and Supplementary Movies 3,4 ), for a 90° Miura pattern with 5 × 5 parallelogram faces, the areal deformability ∈ Areal can be as high as 1,600%, which can be further increased using a denser Miura pattern such as 10 × 10 pattern. It is thus believed that this approach can achieve unprecedented areal deformability compared with all other fabrication methods, to the best of our knowledge. Comparison of origami and conventional LIBs The superior deformability of origami LIBs is mainly due to two mechanisms, namely, the use of rigid origami that can achieve deformability through folding and unfolding at the creases and does not strain the rigid faces, and the use of CNT-coated paper current collectors that survive at the creases and form good adhesive between electrodes. 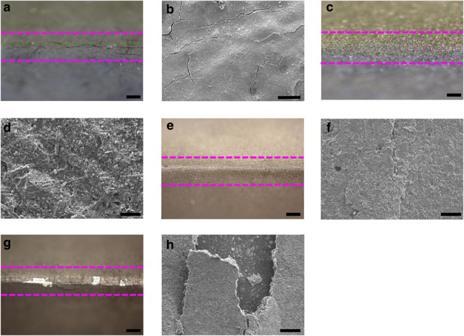Figure 3: Comparison of paper-based origami LIBs with conventional material-based LIBs. For an origami LIB using carbon nanotube (CNT)-coated paper current collectors, after cyclic electrochemical charge and discharge, as well as many cycles of mechanical loads, (a) optical and (b) scanning electron micrographs (SEM) of Li4Ti5O12(LTO) electrodes in the region of a crease as indicated by the magenta dashed lines; (c) optical and (d) SEM images of LiCoO2(LCO) electrodes in the region of a crease as indicated by the magenta dashed lines. (b) and (d) show the entire region of the crease. For an origami LIB using conventional collectors (Cu and Al), after one electrochemical charge and without mechanical loads, (e) optical and (f) SEM images of graphite electrodes on Cu current collector in a region of crease as indicated by the magenta dashed lines; (g) optical and (h) SEM images of LCO electrodes on Al current collector in a region of crease as indicated by the magenta dashed lines. (f) and (h) show the entire region of the crease. Scale bar ina,c,eandgare 2 mm. Scale bar inb,d,fandhare 100 μm. Figure 3a–d shows the optical and SEM images of the lithiated LTO and LCO active layers, respectively, in the regions of a crease, after the cyclic electrochemical characterization and mechanical loads (linear deformation, twisting and bending up to more than 100 times) were performed. Although there were some voids and cracks observed, particularly in the lithiated LTO films at the paper current collector, there was no noticeable delamination from the CNT-coated current collectors as compared with those before lithiation as shown in Supplementary Fig. 1d–g . This behaviour could be explained by the interconnected fabric-like and porous structure of the CNT-coated paper current collectors (as shown in Supplementary Fig. 1a,b ) providing a continuous network for electron transport and significantly enhancing the bonding to the anode and cathode active material layers. To verify this hypothesis, we utilized conventional electrodes and current collectors (that is, graphite on Cu foil for the anode and LCO on Al foil for the cathode) to assemble a LIB cell followed by 45° Miura folding. The assembled LIB cell using conventional materials had a similar thickness (360 μm) as the origami LIBs, and the detailed processes are provided in the supporting information. Supplementary Fig. 7a–d show optical images of the graphite and LCO electrodes before and after folding. It is apparent that some active materials were lost from the conventional current collectors even before charging. Figure 3e–h shows the optical and SEM images of the lithiated graphite and LCO, respectively, in the regions of a crease after the first charge and without mechanical loading. It is now apparent that more electrode materials have been lost, which indicates insufficient thin-film bonding at the creases. Supplementary Fig. 7e shows that the energy capacity of the origami battery using conventional materials decayed about 10% after 100 cycles of linear deformation, in contrast to the steady capacity observations for the origami LIBs using CNT-coated paper current collectors. Therefore, good conductivity and strong bonding after cyclic folding and unfolding are two key attributes for origami LIBs. Figure 3: Comparison of paper-based origami LIBs with conventional material-based LIBs. For an origami LIB using carbon nanotube (CNT)-coated paper current collectors, after cyclic electrochemical charge and discharge, as well as many cycles of mechanical loads, ( a ) optical and ( b ) scanning electron micrographs (SEM) of Li 4 Ti 5 O 12 (LTO) electrodes in the region of a crease as indicated by the magenta dashed lines; ( c ) optical and ( d ) SEM images of LiCoO 2 (LCO) electrodes in the region of a crease as indicated by the magenta dashed lines. ( b ) and ( d ) show the entire region of the crease. For an origami LIB using conventional collectors (Cu and Al), after one electrochemical charge and without mechanical loads, ( e ) optical and ( f ) SEM images of graphite electrodes on Cu current collector in a region of crease as indicated by the magenta dashed lines; ( g ) optical and ( h ) SEM images of LCO electrodes on Al current collector in a region of crease as indicated by the magenta dashed lines. ( f ) and ( h ) show the entire region of the crease. Scale bar in a , c , e and g are 2 mm. Scale bar in b , d , f and h are 100 μm. Full size image The origami design concept enables LIBs with unprecedented mechanical deformability including folding, unfolding, twisting and bending. The use of CNT-coated paper as current collectors provides stable electrochemical characteristics under cyclic mechanical deformations. The fabrication process for origami LIB cells, including slurry mixing, coating and packaging, is completely compatible with mainstream industrial processing. This critical feature of the present work could well benefit the general field of flexible and stretchable electronics from a manufacturability perspective. To utilize this origami battery concept in realistic applications with high level of deformability, at least two approaches can be considered. The first approach would be to build a functional system that includes energy harvesting devices (for example, solar cells), energy storage devices (for example, LIBs) and a functional device (for example, a display) in the same origami platform to enable equivalent deformability to each component in the system. The second approach would be to build a stand-alone LIB by encapsulating the origami battery with highly deformable elastomers to provide a flat device that could then be integrated with other functional devices leading to a fully deformable system. At a high level, the strategy of fusing the art of origami with materials science and energy storage devices provides a markedly alternative approach for powering deformable (including, flexible, foldable, stretchable and curvilinear) electronics ranging from displays, sensors, solar cells and antenna. It is therefore expected that this technology can be applied to various deformable systems. Preparation of origami LIBs on CNT-coated paper CNT-coated paper was prepared as the current collector on laboratory Kimwipes using P3 CNTs from carbon solutions, as described in our previous work [25] . The final mass loading of CNTs on the CNT-coated paper was ~0.8 mg cm −2 . Cathodes and anodes were prepared by depositing LiCoO 2 (LCO, Sigma-Aldrich) and Li 4 Ti 5 O 12 (LTO, MTI Corp.) slurries onto the CNT-coated paper. Multilayer stacking structures as shown in Fig. 1 were prepared with the aluminized polyethylene (PE) (Sigma-Aldrich) as the packaging material, CNT-coated papers as anode and cathode current collectors, LTO and LCO as anode and cathode electrodes, respectively, polypropylene (Celgard 2500) as separator, and 1 M LiPF 6 in EC:DMC:DEC (4:2:4) as electrolyte. The mass ratio for LTO:LCO was fixed at ~1.6. Three layers of anode electrode connected with a copper tab, separator soaked in electrolyte and cathode electrode connected with an aluminium tab were placed in an aluminized/PE bag and assembled in an argon-filled glovebox. Fabrication of origami LIBs using conventional materials Here the same multilayer stacking structures as shown in Fig. 1 were used to fabricate the origami LIBs using the conventional materials, where the aluminized polyethylene (PE) (Sigma-Aldrich) was used as the packaging material, copper (Cu) and aluminium (Al) as the anode and cathode current collectors, respectively, graphite and LCO as anode and cathode electrodes, respectively, polypropylene (Celgard 2500) as separator, and 1 M LiPF 6 in EC:DMC:DEC (4:2:4) as electrolyte. Anode slurries were prepared by mixing graphite (Fisher Scientific), carbon black (Super C45), carboxymethyl cellulose (Fisher Scientific), styrene butadiene rubber (Fisher Scientific) and DI water in a ratio of 76:2:1:2:160 by weight. Then the slurry was uniformly coated on Cu with 20 μm in thickness (CF-T8G-UN, Pred Materials International, Inc.) and then dried on a hot plate at 120 °C for 5 h. Cathode slurries were prepared by mixing LCO, polyvinylidene difluoride (PVDF) (MTI Corp.), carbon black (Super C45) and N-Methyl-2-pyrrolidone solvent (CreoSalus) in a ratio of 18:1:1:20 by weight. Then the slurry was uniformly coated on Al with 10 μm in thickness (Reynolds Wrap) and then dried on a hot plate at 120 °C for 5 h. A mass ratio for graphite:LCO was around 2.0. Then the anode and cathode electrodes were subject to press to make condensed electrodes. Then the same packaging process as discussed in the main text was used. FEA of rigid origami We have developed a non-local model to study the rigid origami that has non-local effects, meaning that each vertex in the origami pattern does not only interact with its nearest-neighboring vertices through the rigid facets, but also interacts with its second-neighboring vertices through dihedral angles between rigid facets. We have implemented this model to a commercial finite element package ABAQUS via its user defined elements. The detailed theory of the mechanics of rigid origami and its finite element implementation will be presented in a separate paper and is out of the scope of the present work. Electrochemical characterization An Arbin electrochemical workstation with a cutoff voltage of 2.65–1.2 V at room temperature was used to conduct cyclic galvanostatic charge and discharge of the origami batteries under folding, unfolding, bending and twisting. Areal coverage was calculated based on the ratio of areas of active electrodes ( L xact × L yact ) and the entire origami battery ( L x × L y ) in the completely unfolded state, as shown in Fig. 2a . The maximum output power of the fully charged battery was calculated using , where V is the open-circuit voltage and R i is the internal resistance as a function of system-level mechanical strain and cycles of mechanical loading. When the origami battery was subjected to different mechanical loading, values of voltage were measured using a voltmeter. The electrochemical impedance spectroscopy (EIS) studies were performed by applying a small perturbation voltage of 5 mV in the frequency range of 0.1 Hz to 100 kHz during the first discharge cycle before and after mechanical deformation, using a Gamry Echem Analyst. The analysis of the impedance spectra was conducted using equivalent circuit software provided by the manufacturer. How to cite this article: Song, Z. et al. Origami lithium-ion batteries. Nat. Commun. 5:3140 doi: 10.1038/ncomms4140 (2014).